Dynamic localization of electronic excitation in photosynthetic complexes revealed with chiral two-dimensional spectroscopy Time-resolved ultrafast optical probes of chiral dynamics provide a new window allowing us to explore how interactions with such structured environments drive electronic dynamics. Incorporating optical activity into time-resolved spectroscopies has proven challenging because of the small signal and large achiral background. Here we demonstrate that two-dimensional electronic spectroscopy can be adapted to detect chiral signals and that these signals reveal how excitations delocalize and contract following excitation. We dynamically probe the evolution of chiral electronic structure in the light-harvesting complex 2 of purple bacteria following photoexcitation by creating a chiral two-dimensional mapping. The dynamics of the chiral two-dimensional signal directly reports on changes in the degree of delocalization of the excitonic states following photoexcitation. The mechanism of energy transfer in this system may enhance transfer probability because of the coherent coupling among chromophores while suppressing fluorescence that arises from populating delocalized states. This generally applicable spectroscopy will provide an incisive tool to probe ultrafast transient molecular fluctuations that are obscured in non-chiral experiments. The handed arrangement of pigments in photosynthetic antenna complexes induces optical chirality, manifested through the difference in absorbance of left- versus right-circularly polarized light. Optical activity provides an exquisite probe of electronic and molecular structure, because of its sensitivity to minute structural details [1] . Microscopically, optical chirality arises from corkscrew-like motion of electrons after excitation belying asymmetric interactions of the electron with its environment [2] , [3] , [4] . Femtosecond and time-resolved measurements of optical activity represent a frontier for understanding functional materials and chemical dynamics [5] , [6] , [7] , [8] . In photosynthetic complexes, transient fluctuations in the protein scaffold cause chiral optical response to change following photoexcitation as the delocalization length of the exciton dynamically contracts [9] , [10] , [11] . However, signal strengths orders of magnitude smaller than the achiral background frustrate attempts to create a complete map correlating chiral response and dynamics. The light-harvesting complex 2 (LH2) of Rhodobacter sphaeroides is the peripheral photosynthetic antenna complex in purple bacteria. Structurally, the complex contains two concentric rings of bacteriochlorophyll a chromophores held in place by non-covalent interactions with the surrounding protein scaffold [12] . The rings are referred to as the B850 and B800 because of their pronounced absorption bands in the near-infrared. Excitations flow from the B800 states into the B850 states on a 700-fs timescale at room temperature [13] . Nine carotenoid chromophores are additionally intertwined through the complex and can act as excitation donors to the bacteriochlorophyll chromophores, with energy transfer proceeding on a sub-100-fs timescale [14] . The electronic structure and energy transfer dynamics of the two rings of chromophores have been intensely studied [15] , [16] , [17] and the precise nature of excitations in the system and their dynamics are currently debated in the literature. In particular, the coherence length (or delocalization length) [18] has been interrogated through a variety of experimental methods [9] , [10] , [19] , [20] . Single-molecule experiments have definitively revealed the delocalized nature of states within the B850 ring arising from the close packing and resultant strong interactions between pigments [21] . The two prominent electronic states within the 850-nm band largely correspond to k =±1 excitations on the B850 ring, which semi-classically correspond to excitations travelling in different directions around the ring [11] . Because of the presence of disorder, higher order k states will additionally be weakly optically active and may contribute to the response. However, interactions between chromophores in the B800 ring are on the order of the disorder in site energies and consequently the electronic structure of these states remains less clear [22] , [23] , [24] , [25] . Here we report a chiral two-dimensional (C2D) mapping that allows us to dynamically probe evolution of chiral electronic structure in the LH2 of purple bacteria following photoexcitation. We observe fast protein motions that induce collapse of the electronic wave packet on a femtosecond timescale and thereby suppress memory of the initial chiral response. The ability of two-dimensional methods to separate energy transfer events into cross peaks allows direct visualization of transfer between delocalized states [24] , [26] . We present two complementary C2D experiments where the chiral sensitivity is incorporated into the pump or probe portion of the excitation pulse sequence. We observe that the relaxation dynamics change for the different chiral experiments, which reflect the complex relaxation dynamics of the delocalized excitons. These experiments are sensitive to the effective size of the delocalized state, which allows us to gain insight into the complex relaxation dynamics. Molecular origins of the chiral response To probe the chiral response of LH2, we use a variant of two-dimensional electronic spectroscopy (2DES) [27] , [28] . In 2DES experiments, a series of three precisely timed femtosecond pulses interrogates the system. By varying the time delay between the first two pulses, two-dimensional frequency–frequency correlation maps can be generated as a function of the waiting time, T , between the second and third pulse. The frequency–frequency maps, interpreted simply, correlate an absorption axis, λ τ , with an emission axis, λ t . By varying the waiting time, we probe dynamics of the system following excitation. Because the experiment involves multiple interactions between the system and the laser field, several unique chiral experiments are possible. By controlling the relative polarization of the incoming pulses, we selectively measure a chiral tensor element while eliminating the stronger achiral contributions [2] , [29] . Formally, our scheme depicted in Fig. 1 yields a spectrum proportional to measuring the difference in nonlinear response after excitation with left- versus right-circularly polarized light [30] . Similar strategies have been experimentally realized in the infrared region of the spectrum for both linear [7] and second-order experiments [29] . 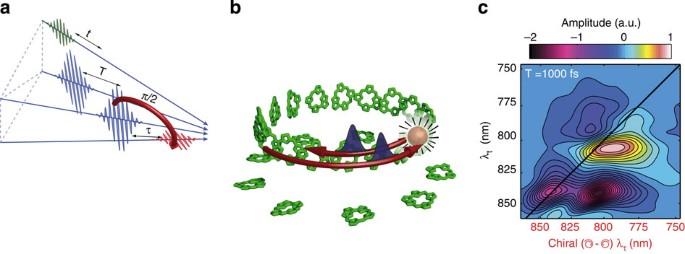Figure 1: Probing chiral wave packet dynamics in LH2. A series of 3 fs laser pulses (a) probe chiral optical response within LH2 using a chirally sensitive polarization scheme. The LH2 complex (b) contains two rings of bacteriochlorophyll a chromophores (phytyl tails and functional groups removed for clarity). Excitations within the inner ring correspond semiclassically to wave packets that travel around the ring in opposing directions, largely corresponding tok=±1. Higher orderkstates will also contribute to the response. Interactions with the surrounding protein leads to scattering events that cause the wave pack to reverse direction. The spectroscopy yields chiral maps (c) of the relaxation dynamics. Figure 1: Probing chiral wave packet dynamics in LH2. A series of 3 fs laser pulses ( a ) probe chiral optical response within LH2 using a chirally sensitive polarization scheme. The LH2 complex ( b ) contains two rings of bacteriochlorophyll a chromophores (phytyl tails and functional groups removed for clarity). Excitations within the inner ring correspond semiclassically to wave packets that travel around the ring in opposing directions, largely corresponding to k =±1. Higher order k states will also contribute to the response. Interactions with the surrounding protein leads to scattering events that cause the wave pack to reverse direction. The spectroscopy yields chiral maps ( c ) of the relaxation dynamics. Full size image Here we probe the chirality of the electronic structure either during the pump sequence or during the probe sequence, which we will refer to as ‘chiral pump’ and ‘chiral probe’. These, respectively, refer to the polarization sequences where the polarization of the first pulse is orthogonal to the subsequent two pulses and signal field for the chiral pump sequence (YXXX), and when the polarization of the third pulse is orthogonal to the other pump pulses and signal field for the chiral probe signal (XXYX). Here the polarization of the three linearly polarized excitation beams and the polarization of the resultant signal are listed in order from left to right (1,2,3, local oscillator/signal). The chiral pump sequence allows us to track differences in the dynamics of initially prepared chiral sub-populations. The chiral probe experiments detect the presence of chiral response following photoexcitation. The resultant signal field from LH2 for both these experiments is three orders of magnitude smaller than the dipole allowed transitions in a typical 2D spectrum of LH2. To detect the weak chiral signal, we use a multiplexed variant of 2DES called GRadient Assisted Photon Echo Spectroscopy (GRAPES) [31] . GRAPES spatially encodes the first time delay across a homogeneous sample to allow two-dimensions of data to be acquired in parallel. The resulting speed-up in acquisition time allows us to average many acquisitions while avoiding noise in the indirect domain, which significantly enhances our signal-to-noise ratio. Complete details of the experimental apparatus and experimental controls can found in the Methods section and accompanying Supplementary Figures . The overall intensity of the signal in an optical activity experiment is related to the rotational strength, which, for many systems (including the LH2 complex) can be expressed as: where is the electric transition dipole moment and is the magnetic transition dipole moment. The helical motion of excitations around the rings of LH2 induces a magnetic transition dipole moment that provides the dominant contribution to the optical activity [2] , [3] , [4] . The precise orientation of the constituent chromophores and their interaction energies dictates the optical response and reproduces the CD spectra of LH2 complexes [32] . Because the chiral signal arises from the corkscrew-like motions of the electrons induced by the strong interactions between chromophores and their environment, these measurements probe the delocalized nature of the electronic structure around the ring. Similarly, superradiance, exchange narrowing, circular dichroism and aspects of the nonlinear optical responses can also report on the degree of delocalization [10] , [20] , [32] , [33] , [34] , [35] . Control experiments conducted on a small dye molecule yielded signal over an order of magnitude smaller than LH2 at similar optical densities, indicating that the predominant contribution to the optical response in LH2 arises from collective excitations (details on the experimental controls can be found in the Methods and Supplementary Information section). Zero waiting time chiral response The experimental results for T =0 fs are shown in Fig. 2 . The C2D maps can be interpreted in a similar manner as the regular 2DES maps, except that in C2D one of the two frequency axes reflects the differential absorbance between left- and right-circularly polarized light. In the absence of dynamics that alters the electronic structure (such as at T =0 fs), we expect the C2D lineshapes along the chiral pump and chiral probe measurement axes in our complementary experiments to coincide, reflecting that the same states are being interrogated. Slices taken through the chiral axis in the 850-nm band at T =0 fs illustrate this effect: a horizontal slice in the chiral pump spectrum and a vertical slice in the chiral probe spectrum match one another. In both cases, we see that the biphasic behaviour characteristic of circular dichroism [1] manifests in the chiral dimension of the 2D map. The two features largely correspond to the k =±1 excitations of the inner B850 ring. Additional contributions from the higher order k states also contribute to this signal. The good agreement between the features at early waiting times verifies the chiral origin of the signal. A similar analysis of the 800-nm feature can be found in Supplementary Fig. 1 . 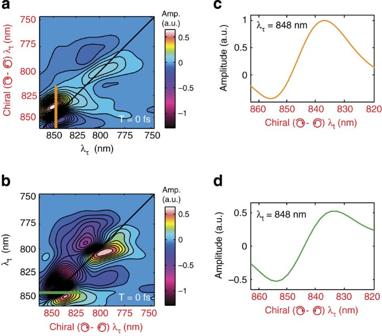Figure 2: Chiral 2D spectra. Chiral two-dimensional (C2D) maps at a waiting timeT=0 fs are shown for the chiral probe (a) and chiral pump (b) polarization sequence. The chiral axes are highlighted in red. Slices through the chiral axis in the 850-nm region, shown by the orange (c) and green (d) traces on the C2D maps, display the characteristic biphasic line shape of linear circular dichroism experiments. The sign of features corresponds to the preferential absorption of left- versus right-circularly polarized light. Figure 2: Chiral 2D spectra. Chiral two-dimensional (C2D) maps at a waiting time T =0 fs are shown for the chiral probe ( a ) and chiral pump ( b ) polarization sequence. The chiral axes are highlighted in red. Slices through the chiral axis in the 850-nm region, shown by the orange ( c ) and green ( d ) traces on the C2D maps, display the characteristic biphasic line shape of linear circular dichroism experiments. The sign of features corresponds to the preferential absorption of left- versus right-circularly polarized light. Full size image Dynamics of chiral response We monitor how optical activity evolves following excitation by acquiring a series of C2D spectra while varying the waiting time. The temporal evolution of the C2D spectral features is displayed in Fig. 3 . C2D spectra at many different waiting times are shown in Supplementary Figs 2 and 3 for the chiral pump and probe experiments. The diagonal features in the chiral pump and chiral probe data show timescales similar to the known energy transfer dynamics, and much of the corresponding dynamics can be rationalized within the current understanding of the disordered exciton model of the electronic dynamics in LH2 (refs 15 , 16 , 17 ). For the chiral pump sequences, we observe a fast 80 fs decay within both the 800- and 850-nm diagonal. Along with the rapid initial decay, the 800-nm feature also shows a slower 600–700 fs decay. Although the 800-nm diagonal feature only broadens and decays, the 850-nm diagonal feature additionally shifts below the diagonal with increasing waiting time, reflecting the known stokes shift of this band [20] . This fast decay component is not present in chiral probe spectra and reflects the internal dynamics of the sub-population of initially prepared chiral states. The fast decay of the 850-nm region has been previously observed and prescribed to localization of the exciton [9] , [18] , [36] , [37] . Localization arises because of excitonic relaxation [37] as well as strong coupling to the bath, which causes the mixing between the excited states to be dependent on the nuclear degrees of freedom [9] , [18] . Concurrent with this fast initial decay, we observe a loss in the biphasic response characteristic of optical activity measurements. The rapid loss of the biphasic response is shown in Fig. 4 . The blue edge of the traces in the 800-nm region for the chiral pump traces arise from energy transfer within the 800-nm band and decay on slower 500–700 fs timescale, whereas the red edge shows a rapid decay. The loss of the biphasic response reflects relaxation and scattering events that cause the memory of the chiral structure to be lost following excitation, resulting from interactions with the protein bath. Semi-classically, the wave packet scatters and reflects thereby losing knowledge of its initial angular momentum. 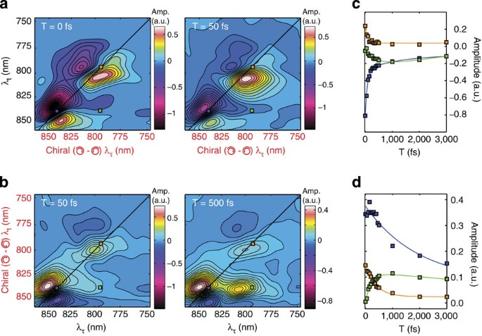Figure 3: Time evolution of C2D spectra. Chiral two-dimensional spectra for the indicated waiting times are shown for the chiral pump (a) and chiral probe (b). Traces through the two main features and the corresponding cross peak are shown incanddfor the chiral pump and chiral probe experiments, respectively. Fits of the traces to a sum of two exponentials are drawn as lines. Amp., amplitude. Figure 3: Time evolution of C2D spectra. Chiral two-dimensional spectra for the indicated waiting times are shown for the chiral pump ( a ) and chiral probe ( b ). Traces through the two main features and the corresponding cross peak are shown in c and d for the chiral pump and chiral probe experiments, respectively. Fits of the traces to a sum of two exponentials are drawn as lines. Amp., amplitude. 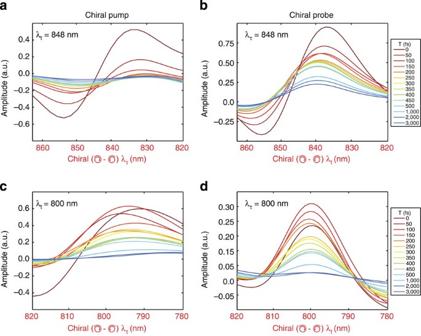Figure 4:Loss of biphasic response. Time evolution of slices through the chiral axis for the chiral pump (a,c) and chiral probe (b,d) for the 850-nm region (a,b) and 800-nm region (b,d). Full size image Figure 4: Loss of biphasic response . Time evolution of slices through the chiral axis for the chiral pump ( a , c ) and chiral probe ( b , d ) for the 850-nm region ( a , b ) and 800-nm region ( b , d ). Full size image At longer waiting times in both sets of C2D spectra, a cross peak appears on the same 500–700 fs timescale observed in traditional 2DES (all-parallel polarization); this feature results from downhill energy transfer between the two rings. The presence of the cross peak in the chiral probe measurement provides direct evidence that the acceptor state in the energy transfer process is delocalized. Energy transfer between the B800 ring and delocalized states on the B850 ring most likely arises from a cooperative excitation energy transfer (supertransfer) mechanism, which is also referred to as generalized Förster theory [24] , [25] , [26] . This collective relaxation process can enhance the energy transfer rate when compared with an incoherent hopping process between localized states [24] , [26] . The enhancement is given by a multiplicative factor proportional to the number of chromophores over which the excitation is delocalized. Although such a delocalized state could arise from mixing instead of through dipolar couplings in generalized Förster theory, no experimental evidence exists for mixing between the electronic states of the B800 and B850 rings. Single-molecule studies on the fluorescent properties of LH2 complexes, which are particularly sensitive to the detailed nature of the electronic states, are well modelled without the inclusion of mixing between excited states of the two rings [21] , [22] . The relaxation process between the rings has been shown to have a coherent contribution that persists at room temperature [38] . Recent single-molecule studies, which are not inhibited by disorder, have further revealed that this coherent contribution lasts for at least 400 fs at ambient temperatures [39] . Furthermore, the single-molecule studies demonstrated weak-field phase control of the excitation energy transfer process, demonstrating that quantum interference effects contribute to the overall transfer efficiency. The precise pathway of energy transfer through LH2 likely varies from complex to complex because of inhomogeneity [25] , [37] , [39] . Such differences are not resolvable with our ensemble measurement. The signal in the 800-nm region is significantly enhanced relative to the 850-nm region in the chiral pump data. This enhancement reflects the higher density of states present in the 800-nm region, arising from both B800 states and higher lying B850* states [25] . Calculations indicate that even though the absorption is roughly equal between the two bands, the density of states in the 800-nm region is roughly twice as large [25] . The signal in the 800-nm region rapidly broadens on an 80-fs timescale, reflecting equilibration of the electronic structure within the B800 chromophores. In the chiral probe data, the 800-nm feature shows a weak but persistent signal that decays on a 340-fs timescale, faster than the 700-fs dynamics observed in the traditional 2DES experiments. Coherences among the B800 chromophores have been measured to dephase on a 180-fs timescale at room temperature in an ensemble measurement [40] . Owing to the inhomogeneity, the coherence lifetime is expected to vary from complex to complex because of the differing shared character and relaxation dynamics of the electronic states [37] , [41] , [42] . The chiral signal may be reporting on a sub-ensemble of more delocalized states, which theory would expect to have enhanced coherence lifetimes. Hence, this decay may report on the collapse of coherence within a sub-ensemble of LH2 complexes. Alternatively, the 340-fs decay could arise from a different physical phenomenon. These data indicate that state coherence within the B800 chromophores cannot be neglected in describing the optical properties of the B800 chromophores. Similarly, the 850-nm diagonal feature decays on a slower 400-fs timescale in the chiral probe data, as can be seen in Figs 3 and 4 . Detailed modelling of the chiral signal will be required to reveal the origin of these slower decays. Chiral spectroscopic measurements provide an incisive tool for studying the structure and dynamics of molecular species. Extension of chiral sensitivity to multidimensional spectroscopy permits direct detection of delocalized states in the B800 band of LH2 at short times. Because of relaxation following photoexcitation, the excitonic wave packet rapidly collapses. Such dynamic localization may have a functional role in the light-harvesting process. Although transfer between collective delocalized states is enhanced because of supertransfer, the corresponding recombination rate of a delocalized state is similarly enhanced. Hence, long-lived delocalized collective excitations would be detrimental to the overall efficiency of transfer because of the increased radiative recombination. The collapse in the size of the acceptor state allows the benefits of enhanced transfer to be realized without the corresponding increase in loss. This method is generally applicable to isotropic media that exhibit a dipolar response, including at infrared wavelengths. Owing to the low signal strength and corresponding long acquisition times, typical circular dichroism experiments only inform about equilibrium configurations [7] . C2D instead probes the change in the chiral structure following photoexcitation, allowing for non-equilibrium photo-activated states to be directly monitored in the visible or infrared. Incorporation of temperature jump [43] or actinic pulses [44] could further drive the system out far of equilibrium to allow for longer timescale conformational changes to be observed. The inherent time resolution of C2D is limited by the lifetime of the free induction decay of the excited state, which is typically on the order of 50 fs at room temperature. The high-temporal resolution and structural resolution provided by C2D makes it an incisive tool for studying photochemical reactions, where fast dynamics and broad spectral line shapes typically complicate their measurement. Spectroscopic apparatus and data analysis Complete details of the GRAPES optical apparatus and laser system has been published previously [31] , [45] . The output of an oscillator seeded regenerative amplifier was focused into a sealed tube of argon at ∼ 1.3 atm, generating a spectrally broadened pulse centred at ∼ 800 nm with ∼ 100 nm full-width at half-maximum. The laser spectrum is shown in Supplementary Fig. 4 , along with the absorption spectrum of LH2. The resultant pulse was compressed using a multi-pulse intrapulse interference phase scan (MIIPS) Box 640 system (Biophotonics Solutions), a spatial light modulator-based pulse shaper, to ∼ 15 fs full-width at half-maximum, as confirmed through a MIIPS scan [46] and TG-FROG [47] measurements preformed at the sample position. The LH2 complex from R. sphaeroides was isolated as previously described [48] . Additional purification was achieved through a DEAE-Sepharose column with 500–600 mM NaCl eluent. The sample concentration used yielded an optical density of ∼ 0.18 at 800 nm in a 200-μm flow cell. The pulse energy was 140 nJ per pulse, resulting in a flux of 42 μJ cm −2 . The GRAPES apparatus was modified by the inclusion of three half-wave plates into beams 1–3, which allows for the complete control of the polarization pulse sequence. The polarization was calibrated at the sample location with a Glan-Thompson polarizer before each experiment, using the polarization of beam 4 as a reference. The extinction ratios for the half-wave plates were measured to be ∼ 10 −5 , which is less than the observed signal strength. Owing to the shallow incoming angles of the four pulses, small contributions from dipole-allowed transitions will also contribute to the response. Separately acquired data on the non-resonant response from fused silica and the laser dye IR144 yielded signals smaller by a factor of ∼ 50 from the signal observed in LH2. Shown in Supplementary Fig. 5 is the all parallel polarization and chiral pump data of the laser dye IR144. In addition, the individual spectra and corresponding dynamics of the chiral response in LH2 are different then the all parallel polarization scheme, which is the leading order contribution of the dipole-allowed response. We thus conclude that the dominant contribution to the signal arises from the chiral tensor elements and not competing dipole-allowed signals. The signal was integrated for 2 s on the charge-coupled device detector and two averages were taken per scan. Relative signal intensities quoted in the text refer to comparisons of the signal intensity, when correcting for differing exposure times, of the phased chiral data and all parallel polarization taken back to back and at the same point in the 2D spectrum. The uncertainty in these numbers is large, as the power stability of our light source is ∼ 0.6% standard deviation over mean, which is significantly greater than the chiral signal. The ability to measure the chiral tensor element independently relieves the need for extremely high-power stability. Scatter subtraction and data analysis proceed as previously described [49] . Images of the processed chiral and all parallel polarization data are shown in Supplementary Fig. 6 with the absolute signal strength. The difference in signal intensity between the chiral and non-chiral data is the same order of magnitude of the difference between the optical absorbance and circular dichroism spectra [32] . To phase the data, separately acquired all parallel polarization data were taken and phased to spectrally resolved transient absorption data [45] , [50] . The pump-probe projections and all parallel 2D spectra are shown in Supplementary Fig. 7 . The 2D spectra are in good agreement with 2D experiments on the related light-harvesting complex 3 (ref. 51 ). The resulting phasing parameters were then used to phase the chiral response, which was taken immediately after the all parallel polarization data. The reported data were qualitatively reproducible on different days with different alignments. How to cite this article: Fidler, A. F. et al. Dynamic localization of electronic excitation in photosynthetic complexes revealed with chiral two-dimensional spectroscopy. Nat. Commun. 5:3286 doi: 10.1038/ncomms4286 (2014).